Effectively suppressing dissolution of manganese from spinel lithium manganate via a nanoscale surface-doping approach The capacity fade of lithium manganate-based cells is associated with the dissolution of Mn from cathode/electrolyte interface due to the disproportionation reaction of Mn(III), and the subsequent deposition of Mn(II) on the anode. Suppressing the dissolution of Mn from the cathode is critical to reducing capacity fade of LiMn 2 O 4 -based cells. Here we report a nanoscale surface-doping approach that minimizes Mn dissolution from lithium manganate. This approach exploits advantages of both bulk doping and surface-coating methods by stabilizing surface crystal structure of lithium manganate through cationic doping while maintaining bulk lithium manganate structure, and protecting bulk lithium manganate from electrolyte corrosion while maintaining ion and charge transport channels on the surface through the electrochemically active doping layer. Consequently, the surface-doped lithium manganate demonstrates enhanced electrochemical performance. This study provides encouraging evidence that surface doping could be a promising alternative to improve the cycling performance of lithium-ion batteries. Owing to their high energy density, lithium-ion batteries (LIBs) are recognized as one of the most appropriate and promising energy-storage systems and are being pursued intensively for transportation applications, including hybrid electric vehicles, plug-in hybrid electric vehicles and pure electric vehicles (PEVs). However, current LIBs do not meet many of the performance and safety requirements for use in PEVs and, therefore, improvements in cell chemistry are being actively pursued to develop a safe and reliable high-performance battery. The cathode is generally regarded as the capacity-determining component of a LIB. Ideally, the cathode should deliver high specific capacity, high operating voltage, low cost, superior safety and long cycle life within a wide working temperature range in order to meet the requirements for PEV applications [1] , [2] . LiMn 2 O 4 with the spinel structure, which shows a reversible Li (de)intercalation plateau at ~4.0 V versus Li/Li + , is one of the most promising cathode materials to meet the above requirements. However, the poor cycling performance of this material, particularly at elevated temperatures, limits its wide application as a cathode material for LIBs [3] . Previous studies [4] , [5] , [6] , [7] , [8] , [9] , [10] , [11] demonstrated that the capacity fade of 4 V LiMn 2 O 4 cells is directly associated with the dissolution of Mn from the cathode/electrolyte interface because of the disproportionation reaction of Mn(III), and the subsequent deposition of Mn 2+ on the anode, thereby increasing the cell impedance. Consequently, suppressing Mn dissolution from the cathode is critical to overcoming capacity fade of the LiMn 2 O 4 cell. One approach to limit the dissolution of Mn from LiMn 2 O 4 is cationic doping on the bulk level, which helps to stabilize the LiMn 2 O 4 crystal structure. The substitution of Mn by cations, such as Al 3+ or Ti 4+ , has been successfully used to minimize capacity fade, but with an inevitable sacrifice of the specific capacity due to the electrochemical inactivity of these dopant ions [12] , [13] , [14] , [15] , [16] . Both cycling performance and capacity can be improved if an electrochemically active cation, for instance, Ni 2+ or Co 2+ , is applied as the dopant. However, such doped LiMn 2 O 4 could lead to safety issues because of the high chemical activity of the doped cations, in particular, Ni 4+ (refs 17 , 18 , 19 ). Another approach that has been widely used to suppress Mn dissolution from LiMn 2 O 4 is to coat the surface, thereby preventing direct contact between the electrolyte and LiMn 2 O 4 . For instance, thin metal oxide coatings on the spinel surface can enhance the resistance of LiMn 2 O 4 against hydrogen fluoride attack from the electrolytes [20] , [21] , [22] , which is the primary mechanism for Mn dissolution. However, uniformity and continuity of the coating layers remain an issue since uncoated portions of the active materials are still subject to electrochemical attack. In some cases, surface-coating does not significantly reduce capacity fade. Another issue with the surface-coating approach is the potential dissimilarity of crystal structures between the coating layer and the active LiMn 2 O 4 spinel material. The heterostructural interface between the coating layer and the active material may lead to phase segregation or separation during cycling of the cell. In addition, the higher resistance imposed by some surface coatings can block ionic and electronic transportation channels on the LiMn 2 O 4 surface [20] , leading to a significant decrease in the cell capacity. In light of the above issues, the present study explores an alternative approach to suppress Mn dissolution from LiMn 2 O 4 and thereby improve the cycling performance of the cell, especially at elevated operating temperature. We propose a nanoscale surface-doping approach to exploit the advantages of both bulk doping and surface-coating techniques while maintaining high capacity, safety, charge transport and cathode stability. In our approach, an electrochemically inactive cation, in this case Ti 4+ , is incorporated only into the surface (a few nanometres thick only) of the spinel LiMn 2 O 4 to form a cation-doped LiMn 2− x Ti x O 4 surface layer, as illustrated in Fig. 1 . This approach exploits the advantage of bulk doping, that is, stabilization of the LiMn 2 O 4 crystal structure throughout the particle. At the same time, the cation-doped surface layer protects the bulk LiMn 2 O 4 from acid corrosion like a surface-coating layer. However, unlike the physical barrier imposed by surface coatings, the LiMn 2− x Ti x O 4 surface layer is electrochemically active and therefore maintains the ion and charge transport channels on the surface. Moreover, the sol–gel method used in this study provides a uniform surface-doped layer over the entire particle and minimizes possible phase segregation owing to the structural similarity between the surface-doped layer (LiMn 2− x Ti x O 4 ) and spinel LiMn 2 O 4 . As a consequence, the surface-doped LiMn 2 O 4 demonstrates significantly enhanced electrochemical performance in terms of cycleability and capacity at elevated temperature. This study suggests that surface doping is a promising alternative approach to improve the cycle performance of the LIBs. 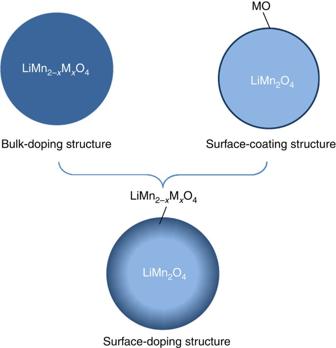Figure 1: Schematic illustration. The structures resulting from bulk- doping, surface-coating and surface-doping (M represents the dopant cation). Figure 1: Schematic illustration. The structures resulting from bulk- doping, surface-coating and surface-doping (M represents the dopant cation). Full size image Characterization of the surface-doping and -coating structures To evaluate our surface-doping approach, two surface modification methods were utilized on pre-synthesized LiMn 2 O 4 , as detailed in the experimental section. In one method, a TiO 2 -surface-doped LiMn 2 O 4 (designated as TSD-LMO hereafter) was prepared using sol–gel technique. In the other approach, TiO 2 -surface-coated LiMn 2 O 4 (designated as TSC-LMO hereafter) was prepared using atomic layer deposition (ALD) [23] . The starting material in both cases consisted of LiMn 2 O 4 particles with a particle size ~200 nm prepared by a conventional solid-state method ( Fig. 2a ). The smooth facets, particle size and octahedral morphology of the unmodified LiMn 2 O 4 particles were unchanged after both the surface-doping ( Fig. 2b ), and ALD-coating ( Fig. 2c ). 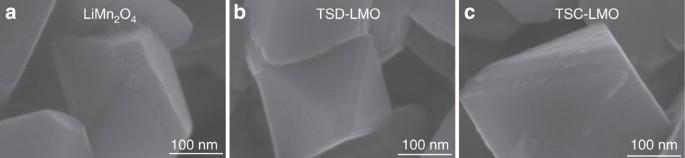Figure 2: Scanning electron microscopy images of particles. (a) Unmodified LiMn2O4, (b) TSD-LMO via sol–gel method and (c) TSC-LMO via ALD (scale bar in all images, 100 nm). Figure 2: Scanning electron microscopy images of particles. ( a ) Unmodified LiMn 2 O 4 , ( b ) TSD-LMO via sol–gel method and ( c ) TSC-LMO via ALD (scale bar in all images, 100 nm). Full size image The crystal structures of the samples were characterized by high-energy X-ray diffraction (XRD) as shown in Fig. 3 . The XRD patterns for all three samples exhibit only the characteristic diffraction peaks for a well-crystallized spinel structure with Fd-3m symmetry. Rietveld refinements of these XRD showed that the TSC-LMO sample has essentially the same lattice parameter as that of the unmodified LiMn 2 O 4 , indicating that the ALD surface-coating does not change the crystal structure of LiMn 2 O 4 , either on the surface or within the bulk. However, in the case of the TSD-LMO sample the lattice parameter is slightly increased compared with the as-synthesized powder. This increase in lattice parameter can be attributed to the diffusion of Ti 4+ ions into the surface spinel lattice by replacing some of the manganese ions of LiMn 2 O 4 during the sol–gel process. The resulting surface-doped LiMn 2− x Ti x O 4 spinel-type layer has a slightly higher lattice parameter because the ionic radius of Ti 4+ is larger than that of the manganese ion [24] , [25] , [26] , [27] . In addition, the absence of TiO 2 peaks in the XRD patterns for the TSC-LMO sample is probably caused by the low concentration or the amorphous state of the ALD TiO 2 . 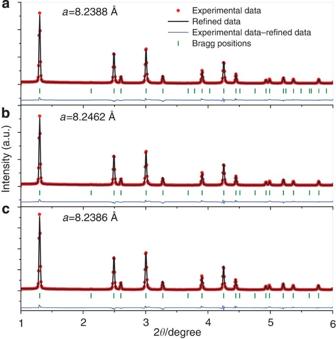Figure 3: XRD patterns and corresponding cubic lattice parameters. (a) Unmodified LiMn2O4, (b) TSD-LMO via sol–gel method and (c) TSC-LMO via ALD. The red dots, black lines, blue lines and green bars represent the experimental data, refined data, their difference and the Bragg positions, respectively. Figure 3: XRD patterns and corresponding cubic lattice parameters. ( a ) Unmodified LiMn 2 O 4 , ( b ) TSD-LMO via sol–gel method and ( c ) TSC-LMO via ALD. The red dots, black lines, blue lines and green bars represent the experimental data, refined data, their difference and the Bragg positions, respectively. Full size image X-ray absorption spectroscopy (XAS) measurements were performed to evaluate the local bonding environment for the Ti and Mn ions in both samples. 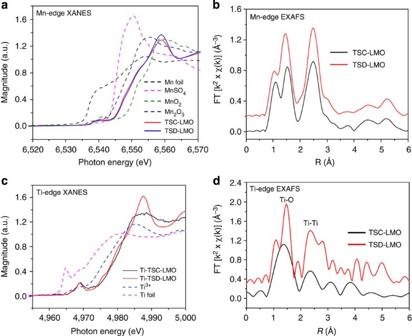Figure 4: X-ray absorption spectroscopy. (a) Mn K-edge XANES, (b) Mn K-edge EXAFS, (c) Ti K-edge XANES, (d) Ti K-edge EXAFS spectra for TSC-LMO (k=2–7.5Å−1) and TSD-LMO (k=1.7–12Å−1) samples. Figure 4a,b shows Mn K-edge XAS spectra for TSC-LMO and TSD-LMO samples. Both surface-modified LiMn 2 O 4 samples exhibit nearly identical features as the unmodified LiMn 2 O 4 in X-ray absorption near edge structure (XANES, Fig. 4a ) and in extended X-ray absorption fine structure ( Fig. 4b ) spectra. These results suggest that the bulk crystal structure of spinel LiMn 2 O 4 is not affected by the surface modifications. The Ti K-edge EXAFS spectra in Fig. 4d , on the other hand, reveal a significant difference of the bonding length of the Ti species on the surface between the TSC-LMO and TSD-LMO samples, although the Ti K-edge XANES data ( Fig. 4c ) showed that Ti is tetravalent in both samples. The Fourier transform for the first shell coordination of the TSC-LMO sample (black curve in Fig. 4d ) has two main peaks: a large peak at ~1.4 Å (uncorrected distance for Ti–O) and a smaller peak at ~2.4 Å (uncorrected distance for Ti–Ti). This spectrum is typical for the K-edge extended X-ray absorption fine structure of TiO 2 . The TSD-LMO sample also shows typical Ti–O and Ti–Ti bonding features (red curve in Fig. 4d ); however, two extra bonding features are also observed (marked as arrow), likely because of either the interactions between Ti and Mn(IV/III) (that is, Ti–Mn 4+ and Ti–Mn 3+ ) or Ti–O bonding with different bond length in the TSD-LMO sample. This can be attributed to the diffusion of Ti 4+ into the surface of the LiMn 2 O 4 particles and the formation of a surface-doped LiMn 2− x Ti x O 4 layer during the calcination process. The XAS results provide further evidence that the TSD-LMO sample has a different surface crystal structure from that of the TSC-LMO sample. Figure 4: X-ray absorption spectroscopy. ( a ) Mn K-edge XANES, ( b ) Mn K-edge EXAFS, ( c ) Ti K-edge XANES, ( d ) Ti K-edge EXAFS spectra for TSC-LMO ( k =2–7.5Å −1 ) and TSD-LMO ( k =1.7–12Å −1 ) samples. Full size image Next, the surface compositions of the samples were examined by X-ray photoelectron spectroscopy (XPS), as shown in Fig. 5 . Ti 2p 1/2 and 2p 3/2 peaks at about 463.8 and 458.2 eV with a spin-orbit splitting of 5.60 eV can be assigned to Ti(IV) ( Fig. 5a ), illustrating the formation of Ti 4+ -containing layers for both the TSC-LMO and TSD-LMO samples, in agreement with the Ti K-edge XANES results. A more distinct difference between the TSC-LMO and TSD-LMO samples can be observed in the Mn 2p spectra shown in Fig. 5b . The TSC-LMO sample exhibits a Mn 2p spectrum similar to the unmodified LiMn 2 O 4 , with the molar ratio of Mn 3+ : Mn 4+ of 1:1. However, in the case of the TSD-LMO sample, the Mn 2p peaks moves toward higher binding energy (by about 0.4 eV), and the molar ratio of Mn 3+ : Mn 4+ is 2:1. This indicates that some of the Mn 4+ cations on the surface of the spinel LiMn 2 O 4 particles have been replaced by Ti 4+ in the TSD-LMO sample, supporting the conclusion that the TSD-LMO sample has a different surface composition compared to the TSC-LMO sample. 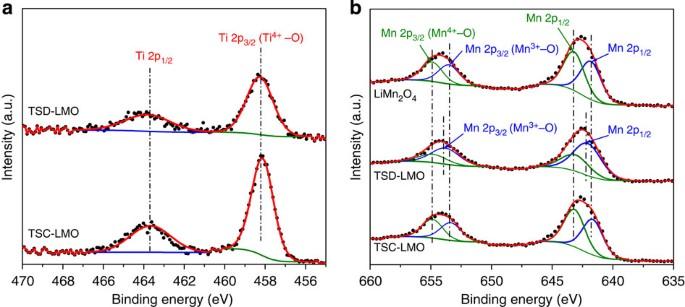Figure 5: X-ray photoelectron spectroscopy. (a) Ti 2p and (b) Mn 2p spectra of unmodified LiMn2O4, TSD-LMO via sol–gel method and TSC-LMO via ALD. The dots and lines represent the experimental data and fitted data, respectively. Figure 5: X-ray photoelectron spectroscopy. ( a ) Ti 2p and ( b ) Mn 2p spectra of unmodified LiMn 2 O 4 , TSD-LMO via sol–gel method and TSC-LMO via ALD. The dots and lines represent the experimental data and fitted data, respectively. Full size image High-resolution transmission electron microscopy (HR-TEM) was used to further investigate the surface morphology and crystallinity of the samples. 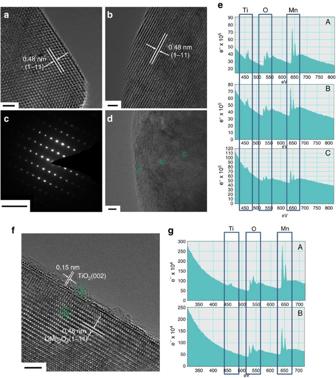Figure 6: High-resolution TEM images of surface-treated LiMn2O4particles. (a,b) High-resolution TEM images of surface-doped LiMn2O4particles showing uniform structure from surface to the interior (scale bar, 2 nm). (c) Selected area diffraction pattern along [112] for the region shown inb. (d) TEM image with regions indicated for the corresponding EELS data shown ine(scale bar, 5 nm). (f) High-resolution TEM image of surface-coated LiMn2O4particle (scale bar, 5 nm). (g) EELS spectra from regions A and B in (f). Figure 6a presents the HR-TEM image for the unmodified LiMn 2 O 4 , showing that the particles are well crystallized with lattice spacing of 4.8 Å, corresponding to the (1–11) spacing of bulk LiMn 2 O 4 and have an atomically smooth surface. After the surface-doping via sol–gel method, the TSD-LMO sample retains the atomically smooth surface and spinel structure, as illustrated in Fig. 6b,c . The presence of Ti in the TSD-LMO surface is confirmed by the electron energy loss spectroscopy (EELS) spectra on different spots of a selected particle ( Fig. 6d,e ). These results indicate that Ti 4+ from the sol–gel precursor diffuses into the LiMn 2 O 4 particle to form a doped layer (LiMn 2− x Ti x O 4 ) on the particle surface during the sol–gel process. Figure 6f shows the HR-TEM image for the TSC-LMO sample, and reveals island-like particles attached to the surface of the LiMn 2 O 4 particles after the ALD coating. These island-like particles have a lattice spacing close to 1.5 Å, consistent with TiO 2 . The HR-TEM ( Fig. 6f ) and EELS from different spots (A and B in Fig. 6g ) of a selected TSC-LMO particle confirm that the ALD TiO 2 exists as a physically distinct phase attached to the LiMn 2 O 4 surface, which is a completely different surface structure from the TSD-LMO sample. Figure 6: High-resolution TEM images of surface-treated LiMn 2 O 4 particles. ( a , b ) High-resolution TEM images of surface-doped LiMn 2 O 4 particles showing uniform structure from surface to the interior (scale bar, 2 nm). ( c ) Selected area diffraction pattern along [112] for the region shown in b . ( d ) TEM image with regions indicated for the corresponding EELS data shown in e (scale bar, 5 nm). ( f ) High-resolution TEM image of surface-coated LiMn 2 O 4 particle (scale bar, 5 nm). ( g ) EELS spectra from regions A and B in ( f ). Full size image The comprehensive characterization described above demonstrates that the sol–gel and ALD approaches for modifying the LiMn 2 O 4 surface yield distinctly different outcomes. In particular, the sol–gel approach generates a continuous surface region enhanced in the electrochemically inactive, and dissolution-resistant Ti 4+ , but without disturbing the spinel crystalline structure that gives rise to high ionic and electronic conductivity. Consequently, this should be beneficial to electrochemical performance in terms of cycleability and capacity, as demonstrated below. Improvement in the electrochemical stability of the spinel cathode The charge/discharge behaviours of the unmodified and surfaced-modified LiMn 2 O 4 electrodes cycled between 3.5 and 4.3 V at 55 °C are compared in Fig. 7 . As shown in Fig. 7a , two plateaus are observed in the charge or discharge curves for all three samples, which can be readily assigned to a one-phase transition reaction at 3.9 V and a two-phase transition reaction at 4.1 V, respectively [28] . Despite differences in the capacities, the unmodified and TSC-LMO electrode exhibited similar charge/discharge curves in shape, while the plateaus for the TSD-LMO electrode were rather different. These differences in the plateau shape can be seen more clearly in the differential capacity versus voltage (d Q /d V versus V ) curves, as shown in Fig. 7b . The oxidation peak at ~4.1 V was significantly broadened in the TSD-LMO electrode, which is likely because of the formation of a LiMn 2− x Ti x O 4 layer on the surface of the LiMn 2 O 4 particles. This layer can subsequently influence the phase transition process because of the change in the crystal structure of the surface. In addition, the initial columbic efficiencies of the TSD-LMO and TSC-LMO (94.9% and 96.1%, respectively) are higher than that of the unmodified LMO (92.3%), indicating that in both cases the surface modification can suppress irreversible reactions (such as deposition of electrolyte decomposition products) on the surface of the cathodes, owing to the stabilized surface structure. 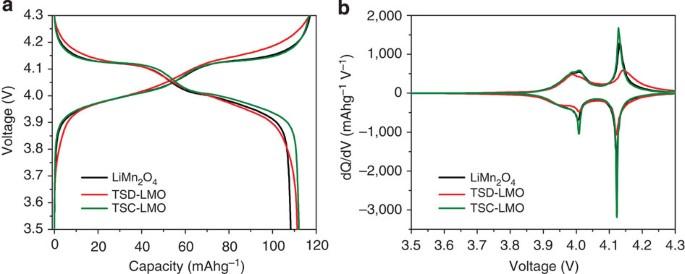Figure 7: The cycle-discharge behaviour analysis. (a) Charge–discharge profile and (b) differential capacity versus voltage curves of the first cycle of the cells with surface-treated and -unmodified LiMn2O4electrodes cycled between 3.5 and 4.3 V at C/10 and 55 °C. Figure 7: The cycle-discharge behaviour analysis. ( a ) Charge–discharge profile and ( b ) differential capacity versus voltage curves of the first cycle of the cells with surface-treated and -unmodified LiMn 2 O 4 electrodes cycled between 3.5 and 4.3 V at C/10 and 55 °C. Full size image The cycling performance of the surface-modified LiMn 2 O 4 samples at elevated temperature (55 °C) is shown in Fig. 8 . Both the TSD-LMO and TSC-LMO samples showed considerably improved cycle performance compared with the unmodified LiMn 2 O 4 . Capacity fade was clearly observed for the unmodified LiMn 2 O 4 cell after 20 cycles and this fade severely accelerated after 70 cycles. By the end of the 100th cycle, the unmodified LiMn 2 O 4 cell had lost almost 60% of its initial capacity. In contrast, the capacity loss of the surface-modified LiMn 2 O 4 (TSD-LMO and TSC-LMO) cells is much lower, indicating that surface modification effectively stabilizes the crystal structure of LiMn 2 O 4 and minimizes Mn dissolution. Moreover, the TSD-LMO electrode shows a higher specific capacity than the TSC-LMO electrode in the same voltage window. This is most likely due to faster Li-ion transfer through the Ti-doped (LiMn 2− x Ti x O 4 ) layer of the TSD-LMO sample compared with transport through the TiO 2 -coating layer of the TSC-LMO samples. To confirm this, we performed electrochemical impedance spectroscopy on the samples after the charge–discharge cycle test. 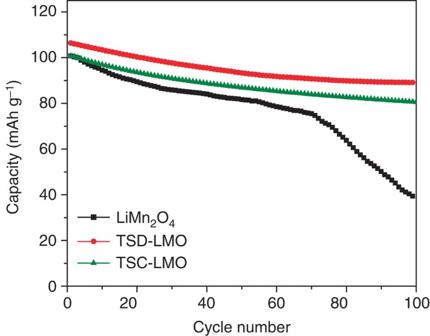Figure 8: Cycling performance. Cycling performance for unmodified LiMn2O4, TSD-LMO via sol–gel deposition and TSC-LMO via ALD, at the rate of C/2 and 55 °C. Figure 8: Cycling performance. Cycling performance for unmodified LiMn 2 O 4 , TSD-LMO via sol–gel deposition and TSC-LMO via ALD, at the rate of C/2 and 55 °C. 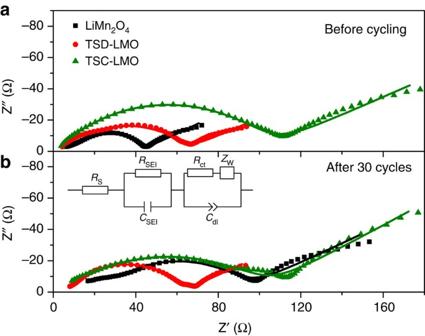Figure 9: Impedance spectra. Impedance spectra (Nyquist plots) of unmodified LiMn2O4, TSD-LMO and TSC-LMO electrodes at 50% DOD (a) during the first discharge and (b) after 30 cycles at 55 °C. The scatter points are the experimental data and the lines represent the simulation results using the equivalent circuit shown in the inset. Full size image Figure 9 shows the AC impedance spectra (Nyquist plots) of the unmodified and surface-modified LiMn 2 O 4 electrodes measured at 50% depth of discharge (DOD) during the first discharge and after cycling at 55 °C. The equivalent circuit shown in the insert of Fig. 8 was used to fit the spectra, where R s is the electrolyte resistance, and R SEI and C SEI are the resistance and geometric capacitance of the anode solid-electrolyte interphase, respectively. R ct reflects the charge-transfer resistance, C dl represents the double-layer capacitance that takes the roughness of the particle surface into account, and Z W is the Warburg diffusional impedance. The semicircle at the high-frequency region of the impedance spectra can be assigned to the R SEI C SEI and R ct C dl elements, while the slope of the low-frequency region is governed by the Warburg diffusion of Li ions from the surface to the centre of the cathode particles [29] , [30] . As shown in Fig. 9a and listed in Table 1 , R ct of the LMO electrode was increased by the surface modification because the surface-doping and -coating layers are not as favourable for Li ion intercalation as the unmodified spinel. However, it is worth noting that R ct for the TSD-LMO electrode (55.3 Ω) is much smaller than that for the TSC-LMO electrode (95.8 Ω), indicating that charge transfer on the surface of the TSD-LMO is faster than that of TSC-LMO. This is because the surface-doping layer maintains the spinel structure of the unmodified LMO for rapid lithium intercalation, while the surface-coating layer by ALD forms a partial physical barrier ( Fig. 6f ) that blocks lithium insertion. Figure 9: Impedance spectra. Impedance spectra (Nyquist plots) of unmodified LiMn 2 O 4 , TSD-LMO and TSC-LMO electrodes at 50% DOD ( a ) during the first discharge and ( b ) after 30 cycles at 55 °C. The scatter points are the experimental data and the lines represent the simulation results using the equivalent circuit shown in the inset. Full size image Table 1 Fitting results for the impedance spectra in Fig. 9 . Full size table Comparing Fig. 9a,b , a remarkable divergence in the impedance change between the unmodified and surface-modified LMO cathodes upon cycling can be observed. The R ct of the unmodified LiMn 2 O 4 electrode more than doubled after 30 cycles, from 4.35 to 11.9 Ω, and the R SEI of the anode increased from 32.8 to 65.4 Ω. The increase in R ct is caused by a structural change of the cathode surface because of Mn dissolution, and the increase in R SEI results from the compositional change of the SEI at the anode due to Mn 2+ deposition [4] , [7] . In contrast, the increase in impedance was negligible for the surface-modified LMO electrodes. Results from inductively coupled plasma-optical emission spectroscopy measurements showed that the concentration of Mn dissolved in the electrolyte decreased from 176 p.p.m. (unmodified LMO cell) to 135 p.p.m. (TSD-LMO cell) [4] and 93 p.p.m. (TSC-LMO cell). Moreover, the concentration of Mn deposited on the anode was 792 p.p.m. for the unmodified LMO cell but only 250 p.p.m. (ref. 4 ) in the TSD-LMO cell and 263 p.p.m. in the TSC-LMO cell. These results clearly demonstrate that surface modification was effective in suppressing the Mn dissolution–migration–deposition process, leading to a negligible impedance rise for both the cathode and anode of the LMO-based cells. As a consequence, the cycling performance of the cells with surface-modified LiMn 2 O 4 electrodes is improved significantly. In our earlier work, we have demonstrated the correlation between Mn deposition (and the consequent impendence rise at the anode) and capacity fading for the same system [4] , which is also consistent to the results presented in this study. In addition, the surface-doping could help to maintain the rate capability of the spinel because of the less increased impedance of the cathode. Finally, it should be pointed out that the Li diffusion path in the bulk of the spinel particles is barely affected by the surface modification as shown by fitting the low-frequency regions of the impedance spectra. These results are detailed in the Methods section. It should be noted that stoichiometric LiMn 2 O 4 has been selected as the cathode material in the current study, since it is the model system for investigating the Mn dissolution phenomenon. However, stoichiometric LiMn 2 O 4 , especially with the nanoscale particle as in this work, is well known to have a severe Mn dissolution issue, which certainly leads to a very fast capacity decay at high temperature. With surface doping, the high-temperature performance of the stoichiometric LiMn 2 O 4 –C cell has been significantly improved, although it still shows capacity degradation upon cycling. More importantly, the main goal of the current study is to find a new alternative approach to the existing surface-coating method to improve the cell performance, as we have demonstrated in this study. In general, we are expecting that the surface-doping technique could also benefit other systems, including layered material such as LiNi x Mn y Co 1− x − y O 2 , Li-rich materials ( x Li 2 MnO 3 ·(1− x )LiMO 2 where M=Mn, Ni, Co, Al, Fe, and so on) and 5 V spinel (LiMn 1.5 Ni 0.5 O 4 ), since they also have the same Mn dissolution issues. In summary, surface modification by ALD or sol–gel treatment has been shown to significantly improve the capacity and cycleability of LiMn 2 O 4 cathodes at elevated temperature. In particular, the uniform surface-doping layer (LiMn 2− x Ti x O 4 ) achieved by sol–gel treatment is favourable for charge transfer since it retains the spinel structure, but it suppresses the dissolution and deposition of manganese by preventing the electrolyte erosion of LiMn 2 O 4 particles. In addition, the surface-doping concept provides advantages over traditional surface-coating techniques because it maintains a continuous surface-to-bulk structure that minimizes phase segregation or separation at interfaces during cycling. These results suggest great opportunities to improve lithium-ion battery performance by optimization of the electrolyte–electrode interphase. Unmodified and modified LiMn 2 O 4 synthesis and characterization Stoichiometric LiMn 2 O 4 particles were synthesized by heating a thoroughly ground mixture of Li 2 CO 3 (Sigma-Aldrich, 99.0%) and chemical MnO 2 (Chemetal, 99.5%; Mole ratio=1.05:4) at 800 °C for 12 h in air. For Ti-surface-doped LiMn 2 O 4 , tetrabutyl titanate (Sigma-Aldrich, 99%) was used as the precursor. Tetrabutyl titanate was first dissolved in ethanol to make a 10% solution, and then the solution was slowly dropped into acetic acid solution (10% acetic acid, 56% ethanol and 34% water) with agitation to get the sol, which was further diluted to 5% by adding ethanol to prevent the aggregation of the colloidal. Then, the LiMn 2 O 4 powders were added into the diluted sol, agitated for 20 min, followed by drying at 80 °C and calcination at 750 °C for 4 h. The TiO 2 –ALD coating was performed in a continuous-flow stainless steel reactor described in detail elsewhere. About 300 mg of the LiMn 2 O 4 powders were carefully spread on a stainless steel tray and a stainless steel mesh cover was clamped over the tray to contain the powder while still providing access to the ALD precursor vapours. The LiMn 2 O 4 powders were held in the reactor at 200 °C under continuous flow of 300 s.c.c.m. ultrahigh-purity nitrogen-carrying gas at 1-torr pressure for 30 min to outgas and achieve thermal equilibrium. The TiO 2 was deposited on the LiMn 2 O 4 particles layer by layer for 10 cycles via alternating exposures to titanium isopropoxide (Sigma-Aldrich, 97%) and deionized water at 200 °C with time sequence 60–120–60–180 s, corresponding to the precursor exposure time, N 2 purge time, co-reactant exposure time and N 2 purge time, respectively. The unmodified and surface-modified LiMn 2 O 4 particles were characterized by high-energy synchrotron XRD, which was carried out at the 11-ID-C beamline of the Advanced Photon Source, Argonne National Laboratory. The XRD patterns were collected in the transmission mode using a Perkin Elmer large area detector. The collected two-dimensional patterns were then integrated into conventional one-dimensional patterns (intensity versus 2 θ ) for final data analysis using the Fit2d software. The XRD Rietveld refinement was carried out using the Fullprof Suite 2012. Samples were analysed by XPS using a Kratos Axis Ultra DLD surface analysis instrument. The base pressure of the analysis chamber during these experiments was 3 × 10 −10 torr, with operating pressures around 1 × 10 −9 torr. Spectra were collected with a monochromatic Al Kα source (1,486.7 eV) and a 300 μ × 700 μ spot size. Photoelectron peak positions were shifted back towards their true values and their peak widths were minimized by flooding the samples with low-energy electrons and ions from the charge neutralizer system on the instrument. Peak position correction was further corrected by referencing the C 1-s peak position of adventitious carbon for a sample (284.8 eV, PHI Handbook of Photoelectron Spectroscopy) and shifting all other peaks in the spectrum accordingly. Fitting was carried out using the programme CasaXPS. Peaks were fit as asymmetric Gaussian/Lorentzians, with 0–30% Lorentzian character. The full-width at half-maximum of all subpeaks was constrained to 0.7–2.0 eV, as dictated by instrumental parameters, lifetime broadening factors and broadening due to sample charging. With this native resolution set, peaks were added and the best fit, using a least-squares fitting routine, was obtained while adhering to the constraints mentioned above. Scanning electron microscopy images were taken on Hitachi S5500 at 0.5 kV. In addition, the TEM images were taken by a field-emission transmission electron microscope (FEI Titan 80–300ST) with a spherical and chromatic aberration imaging corrector working at 80 kV. Spherical and chromatic aberration correction enables the microscope to attain resolution better than 0.1 nm (measured by Young’s fringes) at 80 kV. Electrochemistry tests Cathode electrodes were prepared from mixture of 85% LiMn 2 O 4 powders with or without surface modification, 10% carbon black and 5% polyvinylidene difluoride binder. 1-methyl-2-pyrrolidinone was used to make the mixture into a slurry, which was then casted on an aluminium foil using a 200-μm doctor blade. After drying at 75 °C in air for 4 h and another 12 h under vacuum, the laminates were compressed by a rolling press and then punched into 1.6-cm 2 disk electrodes. 2032 coin cells were assembled with electrodes Celgard 2325 separators and GenII electrolytes (1.2 M LiPF 6 in 3:7 EC-EMC solution) in an Argon-filled glove box. Cycle performance of the spinel cathodes were compared by galvanostatical charge/discharge of the cells between 3.5 and 4.3 V at 55 °C at C/2 (calculated by an anticipated capacity of 120 mAh g −1 for LiMn 2 O 4 spinel). The capacity was calculated with pure LiMn 2 O 4 as an active material. AC impedance spectroscopy of the two-electrode coin cells at 50% DOD during the first discharge or after 30 cycles at 55 °C were collected with an EG&G 273A potentiostat and a Solartron SI1260 Frequency Response Analyzer using a 5-mV stimulating wave, with frequency ranging from 100kHz to 20 mHz. Fitting of the impedance spectra At low-frequency region, the real part of the impedance ( Z ′) is linear to the −1/2 power of the angular frequency ( ω −1/2 ), and the slope is call the Warburg coefficient ( σ ). Using the thin-film model, by solving Fick’s second law the Warburg coefficient can be also expressed as [31] : where R is the ideal gas constant, T is the thermodynamic temperature, F is the Faraday constant, n is the valence, D Li is the diffusion coefficient of the Li ions in the cathode, C is the concentration of the Li + ions and S denotes the contacting area between the active material particles and the electrolyte. For the unmodified LiMn 2 O 4 , TSD-LMO and TSC-LMO electrodes, the specific surface areas are similar because of their similar morphology (as can be seen in Fig. 2 ). Assuming the value of the specific area is A cm 2 g −1 , the values of D Li of the LiMn 2 O 4 calculated from Equation (1) are also listed in Table 1 . The diffusion coefficients of the Li ions in the unmodified and surface-modified LMO are similar, which indicates that the Li diffusion path in the bulk of the spinel particles is barely affected by the surface modification. How to cite this article : Lu, J. et al . Effectively suppressing dissolution of manganese from spinel lithium manganate via a nanoscale surface-doping approach. Nat. Commun. 5:5693 doi: 10.1038/ncomms6693 (2014).